Composite-pulse magnetometry with a solid-state quantum sensor The sensitivity of quantum magnetometer is challenged by control errors and, especially in the solid state, by their short coherence times. Refocusing techniques can overcome these limitations and improve the sensitivity to periodic fields, but they come at the cost of reduced bandwidth and cannot be applied to sense static or aperiodic fields. Here we experimentally demonstrate that continuous driving of the sensor spin by a composite pulse known as rotary-echo yields a flexible magnetometry scheme, mitigating both driving power imperfections and decoherence. A suitable choice of rotary-echo parameters compensates for different scenarios of noise strength and origin. The method can be applied to nanoscale sensing in variable environments or to realize noise spectroscopy. In a room-temperature implementation, based on a single electronic spin in diamond, composite-pulse magnetometry provides a tunable trade-off between sensitivities in the μTHz −1/2 range, comparable with those obtained with Ramsey spectroscopy, and coherence times approaching T 1 . Solid-state quantum sensors attract much attention given their potential for high sensitivity and nano applications. In particular, the electronic spin of the nitrogen-vacancy (NV) colour centre in diamond is a robust quantum sensor [1] , [2] , [3] owing to a combination of highly desirable properties: optical initialization and readout, long coherence times at room temperature ( T 1 >2 ms (refs 4 , 5 ), T 2 0.5 ms (ref. 6 )), the potential to harness the surrounding spin bath for memory and sensitivity enhancement [7] , [8] and biocompatibility [9] . Magnetometry schemes based on quantum spin probes (qubits) usually measure the detuning δω from a known resonance. The most widely used method is Ramsey spectroscopy [10] , which measures the relative phase δωt the qubit acquires when evolving freely after preparation in a superposition state. In the solid state, a severe drawback of this scheme is the short free-evolution dephasing time, T 2 *, which limits the interrogation time. Dynamical decoupling (DD) techniques, such as Hahn-echo [11] or Carr–Purcell–Meiboom–Gill [12] sequences, can extend the coherence time. Unfortunately, such schemes also refocus the effects of static magnetic fields and are thus not applicable for DC magnetometry. Even if δω oscillates with a known frequency (AC magnetometry), DD schemes impose severe restrictions on the bandwidth, as the optimal sensitivity is reached only if the field period matches the DD cycle time [1] . Schemes based on continuous driving are thus of special interest for metrology in the solid state, because they can lead to extended coherence times [13] . Recently, DC magnetometry based on Rabi frequency beats was demonstrated [14] ; in that method, a small detuning along the static magnetic field produces a shift ≈( δω 2 )/(2Ω) of the bare Rabi frequency Ω. Despite ideally allowing for interrogation times approaching T 1 , limiting factors such as noise in the driving field [14] and the bad scaling in δω <<Ω make Rabi-beat magnetometry unattractive. More complex driving modulations [15] can provide not only a better refocusing of driving field inhomogeneities, but also different scalings with δω , yielding improved magnetometry. In this work, we use a novel composite-pulse magnetometry method as a means of both extending coherence times as expected by continuous excitation, and keeping a good scaling with δω , which increases sensitivity. The -rotary-echo (RE) is a simple composite pulse ( Fig. 1a ) designed to correct for inhomogeneities in the excitation field [16] ; here, parametrizes the rotation angle of the half-echo pulse. For ≠2 πk , , RE does not refocus magnetic fields along the qubit quantization axes and can therefore be used for DC magnetometry. For =2 πk , RE provides superior decoupling from both dephasing [17] , [18] , [19] and microwave noise and can be used to achieve AC magnetometry [20] . 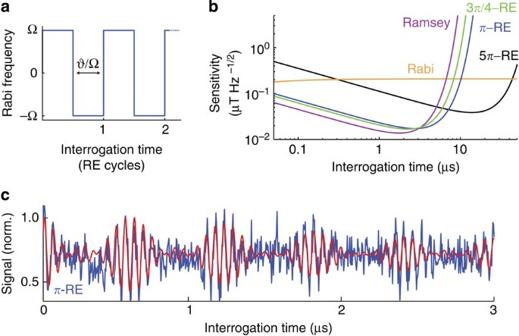Figure 1: RE magnetometry scheme and expected sensitivity. (a) Experimental control composed of an-cycle-RE sequence, in which the phase of the microwave field is switched byπat every pulse of duration/Ω, where Ω is the Rabi frequency. (b) Magnetometry sensitivitiesηREof={3π/4,π, 5π}-RE sequences (green, blue, black), showing the tunability with the half-echo rotation angle. The sensitivity has its global minimumηRE≈1.38/(comparable to Ramsey magnetometry, purple) for≈3π/4 and consecutively increasing local minima for≈(2k+1)π. A decrease in sensitivity is followed by an increase in coherence time, which can approachT1as in Rabi-beat magnetometry (orange), whose sensitivity is limited by Ω. Sensitivities are simulated in the presence of static bath noise using parameters from the fit depicted in (c). (c) A typical normalized fluorescence signal aftern=55 RE cycles for=πand Ω≈2π× 17 MHz (blue); the modulation in the signal is due to the hyperfine interaction with the14N nucleus. The signal is filtered for even harmonics ofπΩ/(mod 2π) (Supplementary Methods) and then fitted to equation (3), modified to include decoherence induced by static bath noise (red). Figure 1: RE magnetometry scheme and expected sensitivity. ( a ) Experimental control composed of a n -cycle -RE sequence, in which the phase of the microwave field is switched by π at every pulse of duration /Ω, where Ω is the Rabi frequency. ( b ) Magnetometry sensitivities η RE of ={3 π /4, π , 5 π }-RE sequences (green, blue, black), showing the tunability with the half-echo rotation angle. The sensitivity has its global minimum η RE ≈1.38/ (comparable to Ramsey magnetometry, purple) for ≈3 π /4 and consecutively increasing local minima for ≈(2 k +1) π . A decrease in sensitivity is followed by an increase in coherence time, which can approach T 1 as in Rabi-beat magnetometry (orange), whose sensitivity is limited by Ω. Sensitivities are simulated in the presence of static bath noise using parameters from the fit depicted in ( c ). ( c ) A typical normalized fluorescence signal after n =55 RE cycles for = π and Ω≈2 π × 17 MHz (blue); the modulation in the signal is due to the hyperfine interaction with the 14 N nucleus. The signal is filtered for even harmonics of π Ω/( mod 2 π ) ( Supplementary Methods ) and then fitted to equation (3), modified to include decoherence induced by static bath noise (red). Full size image Dynamics under RE sequence In the rotating frame associated with the microwave field, and applying the rotating wave approximation, the Hamiltonian describing a continuous stream of -REs is where is the square wave of period T =2 /Ω. On resonance ( δω =0) the evolution is governed by the propagator , with the triangular wave representing the integral of . We approximate the time evolution in the presence of a detuning δω by a first-order Average Hamiltonian expansion [21] of equation (1), yielding an effective Hamiltonian over the cycle ( Supplementary Methods ) Extending the approximation in equation (2) to include the fast Rabi-like oscillations of frequency π Ω/( mod 2 π ), we can thus calculate the population evolution for one of the qubit states, The signal reveals the presence of two spectral lines at for a detuning δω . Sensitivity of the method Thanks to the linear dependence on δω , we expect a favourable scaling of the sensitivity η , given by the shot-noise-limited magnetic field resolution per unit measurement time [1] , [22] . For N measurements and a signal standard deviation , the sensitivity is where γ e (≈2.8 MHzG −1 for NV) is the sensor gyromagnetic ratio and Δ B is the minimum detectable field. We broke down the total measurement time into interrogation time t and the dead-time t d required for initialization and readout. In the absence of relaxation, and neglecting t d , a RE-magnetometer interrogated at complete echo cycles t = n (2 /Ω) yields . As shown in Fig. 1b , RE magnetometry has thus sensitivities comparable to Ramsey spectroscopy, η Ram ≈1/( γ e ). Conversely, Rabi-beat magnetometry has at large times ( Supplementary Methods ), which makes it unsuitable for magnetometry despite long coherence times. To establish the sensitivity limits of RE magnetometry and compare them with other DC-magnetometry strategies, we carried out proof-of-principle experiments in single NV centres in a bulk electronic-grade diamond sample. A static magnetic field B || ≈100 G effectively singles out a qubit {|0 ,|1 } from the NV ground-state spin triplet, as the Zeeman shift lifts the degeneracy between the |±1 levels. The qubit is coupled to the spin-1 14 N nucleus that composes the defect by an isotropic hyperfine interaction of strength A ≈2 π × 2.17 MHz. After optical polarization into state |0 , we apply a stream of n RE cycles using microwaves with frequency ω close to the qubit resonance ω 0 =Δ+ γ e B || , where Δ=2.87 GHz is the NV zero-field splitting. Because of the hyperfine coupling, ω 0 is the resonance frequency only when the nuclear state is m I =0. At room temperature, the nitrogen nucleus is unpolarized and, while its state does not change over one experimental run, in the course of the N ~10 6 experimental realizations, ≈2/3 of the times the qubit is off-resonantly driven by | δω |= A . A typical n -cycle RE fluorescence signal is plotted in Fig. 1c for = π and Ω≈2 π × 17 MHz, while to determine the frequency content of the signal we plot the periodogram ( Supplementary Methods ) in Fig. 2 . 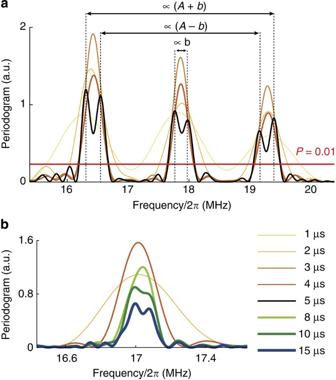Figure 2: The periodogram identifies the frequency content of the signal. (a) Experimental periodogram forπ-RE sequence for increasing interrogation times (thicker lines from 1 to 5 μs, in intervals of 1 μs). The periodogram is defined as the squared magnitude of the Fourier transform of the time signal. A pair of symmetric peaks about the Rabi frequency Ω signals the existence of one detuningδω. The number of resolved frequencies increases with time, at the expense of signal-to-noise ratio. After 5 μs of interrogation, we can estimate both the hyperfine interactionA≈2π× (2.14±0.03) MHz and a small residual detuning from the presumed resonance,b≈2π× (0.17±0.02) MHz. In this estimate, we correct for the real rotation angle≈0.96πusing the difference between the nominal and experimentally realized Rabi frequency (symmetry point in the spectrum). The uncertainty in the measurement is estimated taking into account the total interrogation time, the number of points in the time-domain signal, and the S/N (Supplementary Methods). Periodogram peaks can be tested for their statistical significance33(alsoSupplementary Methods); we confirm that all six frequency peaks are considerably more significant than aP=0.01 significance level (red). (b) Innermost pair of frequency peaks arising from ab≈2π× (64±12) kHz residual detuning in another experimental realization, for an interrogation time of 15 μs. Figure 2: The periodogram identifies the frequency content of the signal. ( a ) Experimental periodogram for π -RE sequence for increasing interrogation times (thicker lines from 1 to 5 μs, in intervals of 1 μs). The periodogram is defined as the squared magnitude of the Fourier transform of the time signal. A pair of symmetric peaks about the Rabi frequency Ω signals the existence of one detuning δω . The number of resolved frequencies increases with time, at the expense of signal-to-noise ratio. After 5 μs of interrogation, we can estimate both the hyperfine interaction A ≈2 π × (2.14±0.03) MHz and a small residual detuning from the presumed resonance, b ≈2 π × (0.17±0.02) MHz. In this estimate, we correct for the real rotation angle ≈0.96 π using the difference between the nominal and experimentally realized Rabi frequency (symmetry point in the spectrum). The uncertainty in the measurement is estimated taking into account the total interrogation time, the number of points in the time-domain signal, and the S/N ( Supplementary Methods ). Periodogram peaks can be tested for their statistical significance [33] (also Supplementary Methods ); we confirm that all six frequency peaks are considerably more significant than a P =0.01 significance level (red). ( b ) Innermost pair of frequency peaks arising from a b ≈2 π × (64±12) kHz residual detuning in another experimental realization, for an interrogation time of 15 μs. Full size image The number of distinguishable frequencies increases with interrogation time at the expense of signal-to-noise ratio. RE magnetometry not only discriminates the frequency shifts due to the hyperfine interaction (we find A ≈2 π × (2.14±0.03) MHz but, for interrogation times as short as 5 μs, it also reveals a small residual detuning b ≈2 π × (0.17±0.02) MHz from the presumed resonance. In contrast, under the same experimental conditions, Rabi magnetometry does not discern such a detuning before an interrogation time ≈188 μs ( Supplementary Methods , and Supplementary Fig. S1 ). With longer interrogation times ~15 μs as in Fig. 2b (also in Supplementary Fig. S2 ), RE can detect a frequency as small as b ≈2 π × (64±12) kHz. To determine the experimental sensitivities, we estimate by driving the qubit with varying ω , at fixed interrogation times t ( Fig. 3a ). For each t , in Fig. 3b we plot the minimum and compare it with the adjusted theoretical sensitivity η /( C × C A ). Here, ( C × C A )≈(5.9±1.4) × 10 −3 in our setup, is a factor taking into account readout inefficiencies and a correction for the presence of the hyperfine interaction [1] (see also Supplementary Methods ). The sensitivities agree with the theoretical model, with optimal ~10 μTHz −1/2 , which is within the range of sensitivities achieved with other magnetometry schemes alternative to Ramsey [23] , [24] , and with the added flexibility made possible by a suitable choice of RE rotation angle. Improved sensitivities are expected from isotopically purified diamond [25] ; an adequate choice of interrogation times or polarization of the nuclear spin can easily set C A =1, while C can be improved by efficient photon collection [26] or using repeated readout methods [27] . 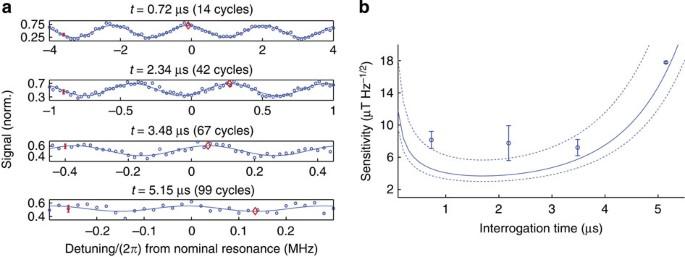Figure 3: Experimental sensitivity of RE magnetometry. (a) RE signals at fixed interrogation times, indicated on top of each sub panel, as a function of the detuningδωfrom resonance. The signals are used to numerically calculateand thus obtain the sensitivityη, given by equation (4). With increasing interrogation times, the slopes initially increase, indicating an improvement inη; the effect of decoherence for the longer interrogation times degrades the sensitivity, and the slopes smoothen accordingly. The different amplitude modulations are due to the three frequencies in the signal, {b,A±b}; polarizing the nuclear spin34would eliminate this modulation. From the fitted resonances for each curve (red diamonds), we estimate the true resonance to be at 0.09±0.15 MHz from the presumed resonance. Typical s.d. in the measurement are indicated (red error bars). Interrogation times are chosen to coincide with minima of the sensitivity in the presence of the hyperfine interaction; in other words, the correction factorCAis at a local maximum at those times (Supplementary Methods, andSupplementary Fig. S3). (b) For each fixed interrogation time, we plot the minimum sensitivityηwithin one oscillation period of the fitted oscillation frequency obtained in (a),τ=2tsin(/2)/(Supplementary Methods, andSupplementary Fig. S4a). The experimental points agree in trend with the theoretically expected sensitivitiesη/(C×CA) (solid curves), here corrected for the presence of static bath noise,.was computed using aT2*≈2.19±0.15 μs fitting from a Ramsey decay experiment (Supplementary Fig. S4b). The dashed blue lines indicate the lower (higher) bounds for the sensitivity estimated by dividing the theoretical sensitivity by the maximum (minimum)C×CAvalue in the set of points. The s.d. is shown in the error bar for each point. Figure 3: Experimental sensitivity of RE magnetometry. ( a ) RE signals at fixed interrogation times, indicated on top of each sub panel, as a function of the detuning δω from resonance. The signals are used to numerically calculate and thus obtain the sensitivity η , given by equation (4). With increasing interrogation times, the slopes initially increase, indicating an improvement in η ; the effect of decoherence for the longer interrogation times degrades the sensitivity, and the slopes smoothen accordingly. The different amplitude modulations are due to the three frequencies in the signal, { b , A ± b }; polarizing the nuclear spin [34] would eliminate this modulation. From the fitted resonances for each curve (red diamonds), we estimate the true resonance to be at 0.09±0.15 MHz from the presumed resonance. Typical s.d. in the measurement are indicated (red error bars). Interrogation times are chosen to coincide with minima of the sensitivity in the presence of the hyperfine interaction; in other words, the correction factor C A is at a local maximum at those times ( Supplementary Methods , and Supplementary Fig. S3 ). ( b ) For each fixed interrogation time, we plot the minimum sensitivity η within one oscillation period of the fitted oscillation frequency obtained in ( a ), τ =2 t sin( /2)/ ( Supplementary Methods , and Supplementary Fig. S4a ). The experimental points agree in trend with the theoretically expected sensitivities η /( C × C A ) (solid curves), here corrected for the presence of static bath noise, . was computed using a T 2 *≈2.19±0.15 μs fitting from a Ramsey decay experiment ( Supplementary Fig. S4b ). The dashed blue lines indicate the lower (higher) bounds for the sensitivity estimated by dividing the theoretical sensitivity by the maximum (minimum) C × C A value in the set of points. The s.d. is shown in the error bar for each point. Full size image Effect of noise The sensitivity of a NV magnetometer is ultimately limited by the interaction of the quantum probe with the nuclear spin bath. We model the effect of the spin bath by a classical noise source along σ z (ref. 28 ), described by an Ornstein–Uhlenbeck (OU) process of strength σ and correlation time τ c . In the limit of long τ c (static bath), the dephasing time associated with RE (Ramsey) magnetometry is ( ) respectively (for the general case, see Supplementary Methods , and Supplementary Fig. S5a ). Although at the optimum interrogation time T ′/2 one has , RE magnetometry allows a greater flexibility in choosing the effective coherence time, as larger ν increase the resilience to bath noise. Thus, one can match the RE interrogation time to the duration of the field one wants to measure. In addition, RE can yield an overall advantage when taking into consideration the dead-time t d . If , as in repeated readout methods [27] , a gain in sensitivity can be reached by exploiting the longer interrogation times enabled by RE magnetometry ( Supplementary Methods , and Supplementary Fig. S6 ). An even larger advantage is given by AC magnetometry with 2 πk -RE [20] , as RE provides better protection than pulsed DD schemes [17] , [20] . Excitation field instabilities along σ x also accelerate the decay of RE and Rabi signals. However, provided the echo period is shorter than τ c , RE magnetometry corrects for stochastic noise in Rabi frequency ( Supplementary Methods , and Supplementary Fig. S5b ). This protection was demonstrated experimentally by applying static and OU noise ( τ c ≈200 ns) in the excitation microwave, both with strength 0.05 Ω. The results for Rabi and ={ π , 5 π }-RE sequences in Fig. 4 clearly show that whereas the Rabi signal decays within ≈0.5 μs, 5 π -RE refocuses static excitation noise and presents only a very weak decay under finite-correlation noise after much longer interrogation times ≈3 μs, in agreement with the theoretical prediction; π -RE is robust against the same noise profiles. 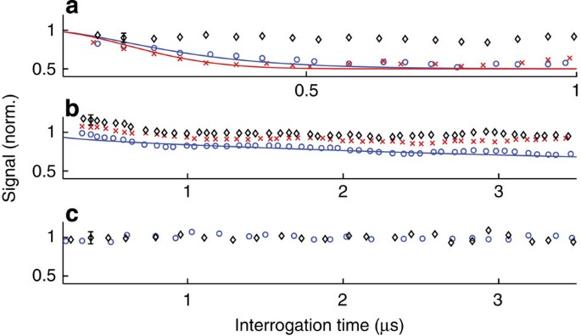Figure 4: The RE is robust against added microwave frequency noise. Forty realizations of both static (red) and Ornstein–Uhlenbeck (OU,τc=200 ns, blue) microwave noise of strength 0.05 Ω, where Ω≈2π× 19 MHz is the Rabi frequency, for (a) Rabi, (b) 5π-RE and (c)π-RE sequences. We note that the correlation time of the driving field noise was purposely set much shorter than what usually observed in experiments in order to enhance the different behaviour ofπ-RE and 5π-RE. Typical s.d. in the measurement are indicated (black error bars). (a) We plot the peak of the Rabi fringes in the presence of static (red crosses) and OU (blue circles) microwave noise, which are in agreement with the expected theoretical decay (solid blue line and solid red line, respectively) (Supplementary MethodsandSupplementary Fig. 5b). The oscillations at the tail of the signals are due to the finite number of experimental realizations. The peaks of a no-noise Rabi experiment are plotted for comparison (black diamonds). (b) The peak of the 5π-RE revivals are plotted in the presence of static (red crosses) and OU (blue circles) microwave noise; the peaks of the 5π-RE in the absence of microwave noise are also plotted for comparison (black diamonds). Although the echo virtually does not decay in the presence of static noise, under the effect of stochastic noise, the echo decays only weakly as stipulated by theory (solid blue line) (Supplementary MethodsandSupplementary Fig. 5b). (c) The peak of theπ-RE revivals are plotted in the presence of OU microwave noise (blue circles); virtually no decay is found if compared with the peaks of a no-noise experiment (black diamonds). Figure 4: The RE is robust against added microwave frequency noise. Forty realizations of both static (red) and Ornstein–Uhlenbeck (OU, τ c =200 ns, blue) microwave noise of strength 0.05 Ω, where Ω≈2 π × 19 MHz is the Rabi frequency, for ( a ) Rabi, ( b ) 5 π -RE and ( c ) π -RE sequences. We note that the correlation time of the driving field noise was purposely set much shorter than what usually observed in experiments in order to enhance the different behaviour of π -RE and 5 π -RE. Typical s.d. in the measurement are indicated (black error bars). ( a ) We plot the peak of the Rabi fringes in the presence of static (red crosses) and OU (blue circles) microwave noise, which are in agreement with the expected theoretical decay (solid blue line and solid red line, respectively) ( Supplementary Methods and Supplementary Fig. 5b ). The oscillations at the tail of the signals are due to the finite number of experimental realizations. The peaks of a no-noise Rabi experiment are plotted for comparison (black diamonds). ( b ) The peak of the 5 π -RE revivals are plotted in the presence of static (red crosses) and OU (blue circles) microwave noise; the peaks of the 5 π -RE in the absence of microwave noise are also plotted for comparison (black diamonds). Although the echo virtually does not decay in the presence of static noise, under the effect of stochastic noise, the echo decays only weakly as stipulated by theory (solid blue line) ( Supplementary Methods and Supplementary Fig. 5b ). ( c ) The peak of the π -RE revivals are plotted in the presence of OU microwave noise (blue circles); virtually no decay is found if compared with the peaks of a no-noise experiment (black diamonds). Full size image The unique ability of the RE-magnetometer to adjust its response to distinct noise sources is relevant when the sample producing the magnetic field of interest is immersed in a realistic environment; moreover, the field source might itself have a finite duration or duty cycle. Most experimentally relevant fields, such as those arising from biological samples, might last only for a finite amount of time, when triggered, or be slowly varying so that one can only record their time-average. Thus, it becomes interesting to be able to tune the interrogation time in order to capture and average over the complete physical process. The advantage is two-fold: the protection from noise can be tuned by changing the echo angle, thus allowing the interrogation times to be varied. Techniques for repeated readout in the presence of a strong magnetic field 1,000 G (ref. 27 ) (also Supplementary Methods ) can at once improve sensitivities and enable the use of much lower qubit resonance frequencies ~MHz, preferable in biological settings. Additionally, a RE-magnetometer can discriminate magnetic noise sources given the sensor’s well-understood decoherence behaviour under different noise profiles, effectively enabling noise spectroscopy for both σ z and σ x -type noises. NV centre-based RE magnetometry could find useful application, for example, to sense the activity of differently-sized calcium signalling domains in living cells, more specifically in neurons. Transient calcium fluxes regulate a myriad of cell reactions [29] . The signalling specificity of such fluxes is determined by their duration and mean travelled distance between membrane channel and cytoplasm receptor. The smaller, faster-signalling domains have resisted thorough investigation via both diffraction-limited optical microscopy [29] , and the use of fluorescing dyes, which do not respond fast or accurately enough to Ca 2+ transients [30] . The magnetic field produced by as few as 10 5 Ca 2+ , being diffused within ~10 μs through a ~200-nm domain, can be picked up by a nanodiamond scanning sensor [31] , [32] with sensitivity ~10 μTHz −1/2 placed at close proximity ~10 nm ( Supplementary Methods ). The trade-off between sensitivity and optimal interrogation time under RE magnetometry can be optimized to the characteristics of the signalling domain under study by a suitable choice of . In conclusion, we have demonstrated a quantum magnetometry scheme based on composite pulses. Its key interest stems both from the continuous-excitation character, offering superior performance for solid state sensors such as the NV centre, and from the possibility of tuning the sensor’s coherence time and sensitivity in the presence of variable or unknown sensing environments, to protect from or map noise sources. Current technology enables immediate implementation of such scheme at the nanoscale. Quantum magnetometer description The NV centre is a naturally occurring point defect in diamond, composed of a vacancy adjacent to a substitutional nitrogen in the carbon lattice. The ground state of the negatively charged NV centre is a spin triplet with zero-field splitting Δ=2.87 GHz between the m S =0 and m S =±1 sub-levels. Coherent optical excitation at 532 nm promotes the quantum state of the defect non-resonantly to the first orbital excited state. Although the m S =0 state mostly relaxes with phonon-mediated fluorescent emission (≈650–800 nm), the m S =±1 states have in addition an alternative, non-radiative decay mode to the m S =0 state via metastable singlet states. Owing to this property, each ground state is distinguishable by monitoring the intensity of emitted photons during a short pulse of optical excitation. Additionally, continuous optical excitation polarizes the NV into the m S =0 state. We apply a magnetic field (≈100 G) along a crystal axis 111 to lift the degeneracy between the m S =±1 states and drive an effective two-level system m S ={0,1} at the resonant frequency ( ω 0 ≈3.15 GHz) obtained by continuous wave electron spin resonance and Ramsey fringe experiments. Experimental setup description Experiments were run at room-temperature with single NV centres from an electronic-grade single crystal plate ([100] orientation, Element 6) with a substitutional nitrogen concentration <5 ppb. The fluorescence of single NV centres is identified by a home-built confocal scanning microscope. The sample is mounted on a piezo stage (Nano-3D200, Mad City Labs). The excitation at 532 nm is provided by a diode-pumped laser (Coherent Compass 315M), and fluorescence in the phonon sideband (~650–800 nm) is collected by a X100, NA=1.3 oil immersion objective (Nikon Plan Fluor). The fluorescence photons are collected into a single-mode broadband fibre of NA=0.12 (Font Canada) and sent to a single-photon counting module (SPCM-AQRH-13-FC, Perkin Elmer) with acquisition time 100 or 200 ns. Laser pulses for polarization and detection are generated by an acousto-optic modulator with rise time 7 ns (1250C-848, Isomet). A signal generator (N5183A-520, Agilent) provides microwave fields to coherently manipulate the qubit. An arbitrary waveform generator at 1.2 GS/s (AWG5014B, Tektronix) is employed to shape microwave pulses with the help of an I/Q mixer (IQ-0318L, Marki Microwave), and to time the whole experimental sequence. Microwaves are amplified (GT-1000A, Gigatronics) and subsequently delivered to the sample by a copper microstrip mounted on a printed circuit board, fabricated in MACOR to reduce losses. A static magnetic field is applied by a permanent magnet (BX0X0X0-N52, K&J Magnetics) mounted on a rotation stage, which in turn is attached to a three-axis translation stage; this arrangement enables the adjustment of the magnetic field angle with respect to the sample. The magnetic field is aligned along a [111] axis by maximizing the Zeeman splitting in a CW ESR spectrum. In each experimental run, we normalize the signal with respect to the reference counts from the m S ={0,1} states, where the transfer to state m S =1 is done by adiabatic passage. How to cite this article: Aiello, C. D. et al . Composite-pulse magnetometry with a solid-state quantum sensor. Nat. Commun. 4:1419 doi: 10.1038/ncomms2375 (2013).